Activity-dependent regulation of dendritic growth and maintenance by glycogen synthase kinase 3β Activity-dependent dendritic development represents a crucial step in brain development, but its underlying mechanisms remain to be fully elucidated. Here we report that glycogen synthase kinase 3β (GSK3β) regulates dendritic development in an activity-dependent manner. We find that GSK3β in somatodendritic compartments of hippocampal neurons becomes highly phosphorylated at serine-9 upon synaptogenesis. This phosphorylation-dependent GSK3β inhibition is mediated by neurotrophin signalling and is required for dendritic growth and arbourization. Elevation of GSK3β activity leads to marked shrinkage of dendrites, whereas its inhibition enhances dendritic growth. We further show that these effects are mediated by GSK3β regulation of surface GABA A receptor levels via the scaffold protein gephyrin. GSK3β activation leads to gephyrin phosphorylation to reduce surface GABA A receptor clusters, resulting in neuronal hyperexcitability that causes dendrite shrinkage. These findings thus identify GSK3β as a key player in activity-dependent regulation of dendritic development by targeting the excitatory–inhibitory balance of the neuron. Elaborate dendritic arbours are a key feature of polarized neurons in the vertebrate brain, and they function in reception, integration and computation of various synaptic inputs [1] . Proper growth, patterning and maintenance of dendritic arbours are essential for normal brain development and function. Intrinsic and extrinsic signals are known to work in concert to generate and maintain the distinct patterns of dendritic arbours of different neuronal types [2] , [3] , [4] . Among them, neuronal activity has a crucial role in dendrite development and maintenance [2] , [5] , [6] , [7] . However, the effects of neuronal activity on dendritic arbours appear to be complex and depend on the nature of the activity, its spatiotemporal patterns, the specific brain regions, as well as particular developmental stages [2] , [5] , [6] , [7] . The mechanisms underlying activity-dependent effects on dendrites remain to be fully elucidated. Given that dendritic arbours are the primary determinant of circuitry wiring and function, it is no surprise that abnormalities in dendritic arbours are associated with a large number of neurological disorders [8] , [9] . Therefore, there is immense interest in understanding the molecular and cellular mechanisms that govern and regulate dendritic development and maintenance. Glycogen synthase kinase 3β (GSK3β) is a serine/threonine kinase that is involved in a wide array of neuronal functions, including Wnt/β-catenin signalling, proteasomal degradation, microtubule dynamics, receptor trafficking, synaptic plasticity, neuronal polarity and axon growth [10] , [11] . GSK3β is highly expressed in the central nervous system, especially in the hippocampus during brain development [12] . However, elevated GSK3β activity has been linked to a number of neurological diseases [13] , [14] , [15] , [16] , [17] , [18] . GSK3β activity is regulated by phosphorylation: phosphorylation of tyrosine-216 leads to activation, whereas phosphorylation of serine-9 results in inhibition [10] , [17] . In cells, inhibition by serine-9 phosphorylation is believed to be the primary mechanism of regulating GSK3β activity. However, because GSK3β determines the output of numerous signalling cascades, it remains a challenge to understand how GSK3β generates diverse effects on neuronal development and function. GSK3β is known to have a crucial role in the establishment of neuronal polarity. Local inhibition of GSK3β is required for the acquisition of axonal identity, whereas GSK3β remains highly active in neighbouring minor (dendritic) processes [19] , [20] . Here we investigated whether GSK3β has a role in dendrite development and maintenance, after the establishment of neuronal polarity. We show that GSK3β is inhibited by neurotrophin signalling in dendrites of cultured hippocampal neurons upon synaptogenesis. Importantly, such GSK3β inhibition is essential for dendritic growth and stabilization. Finally, we identify GABA A receptors (GABA A Rs) as the main target of GSK3β in activity-dependent regulation of dendritic development. Our results reveal a novel role for GSK3β in activity-dependent regulation of dendrite development and maintenance. Inhibition of GSK3β promotes dendrite development Hippocampal neurons in culture develop their axon-dendrite polarity within the first 5 days in vitro (DIV) [21] . Synaptic connections of cultured hippocampal neurons start to form around DIV7–9, peak around DIV11–14 and become relatively stable after 3 weeks [22] , [23] , [24] . To study changes in GSK3β activity at different developmental stages, we examined the level and distribution of phospho-serine-9-GSK3β (pS9-GSK3β) in cultured rat hippocampal neurons at DIV3, 9, 16 and 22. Cells were double labelled with a pan-specific antibody to determine the total levels of GSK3β (Total-GSK3β). To quantify changes in pS9-GSK3β signals, background-subtracted images were normalized to Total-GSK3β to generate ratiometric images depicting the pS9/Total-GSK3β intensity ratio. Consistent with previous studies [19] , we found that pS9-GSK3β was highly concentrated at the tip of axons at DIV3 (arrows; Fig. 1a ), whereas Total-GSK3β signals were relatively uniform ( Fig. 1a , see also Supplementary Fig. S1a ). 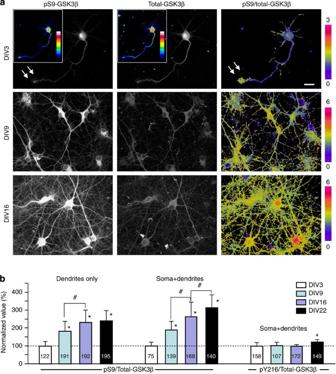Figure 1: Spatiotemporal patterns of pS9-GSK3b in hippocampal neurons in culture. (a) Representative immunofluorescence images of hippocampal neurons from different culture days showing the spatial pattern of pS9-GSK3β (left), total-GSK3β (middle) and their ratios (right). The pS9/Total-GSK3β ratio is depicted in pseudocolors. Colour insets in the DIV3 panels show the immunofluorescence in 16 pseudocolors for better illustration of the spatial distribution of pS9 and total-GSK3β immunofluorescence. Arrows indicate the growth cone of an axon with a high level of pS9-GSK3β fluorescence and pS9/Total-GSK3β ratio. Scale bar,10 μm. (b) Bar graphs showing the quantitative results on the changes in the pS9/Total-GSK3β ratio in the dendrites or soma+dendrites at different days in culture. All data are normalized to the DIV3 average. Numbers indicate the total number of cells examined (from at least three independent batches of culture). Error bars: s.d. *P<0.05 (comparing with DIV3),#P<0.05 (comparing with the indicated group) using Student’st-test. Figure 1: Spatiotemporal patterns of pS9-GSK3b in hippocampal neurons in culture. ( a ) Representative immunofluorescence images of hippocampal neurons from different culture days showing the spatial pattern of pS9-GSK3β (left), total-GSK3β (middle) and their ratios (right). The pS9/Total-GSK3β ratio is depicted in pseudocolors. Colour insets in the DIV3 panels show the immunofluorescence in 16 pseudocolors for better illustration of the spatial distribution of pS9 and total-GSK3β immunofluorescence. Arrows indicate the growth cone of an axon with a high level of pS9-GSK3β fluorescence and pS9/Total-GSK3β ratio. Scale bar,10 μm. ( b ) Bar graphs showing the quantitative results on the changes in the pS9/Total-GSK3β ratio in the dendrites or soma+dendrites at different days in culture. All data are normalized to the DIV3 average. Numbers indicate the total number of cells examined (from at least three independent batches of culture). Error bars: s.d. * P <0.05 (comparing with DIV3), # P <0.05 (comparing with the indicated group) using Student’s t -test. Full size image When hippocampal neurons were examined under identical conditions at either DIV9 or DIV16, we found that pS9-GSK3β levels were markedly increased in the somatodendritic region ( Fig. 1a and Supplementary Fig. S1b ). Quantitative analysis showed that the pS9/Total-GSK3β ratio in the somatodendritic region at DIV9 is 188.69±49.61% (mean±s.d., n =139) of the DIV3 value, and even higher in the hippocampal neurons of later stages ( Fig. 1b ). We confirmed the increase in pS9 levels at DIV9 and 16 using western blot ( Supplementary Fig. S2 ). Conversely, phospho-tyrosine-216 GSK3β levels did not change over the same period (except at DIV22 when a small increase was observed). In addition, at DIV14–16, pS9-GSK3β staining was more intense in dendrites than in axons ( Supplementary Fig. S1c,d ). As DIV9 corresponds to the early stage of synaptogenesis, our findings suggest that the increase in pS9-GSK3β in dendrites may be associated with synapse formation. Because neurotrophin signalling has been associated with synaptogenesis and dendritic development [25] , we tested if it was involved in the elevation of pS9-GSK3β levels in dendrites. We found that inhibition of Trk receptors by the selective inhibitor K252a (ref. 26 ), but not the ineffective analogue K252b, for 2 days (DIV14 to DIV16) resulted in a marked reduction in pS9-GSK3β levels in the somatodendritic region of cultured hippocampal neurons (54.97±8.93% (mean±s.d., n =362) of the control, Fig. 2a ). Correspondingly, bath application of brain-derived neurotrophic factor (BDNF) to DIV14 hippocampal neurons for 2 days further elevated the pS9-GSK3β level in the somatodendritic compartment to 127.99±26.39% (mean±s.d., n =153) of the control ( Fig. 2a ). These results suggest that neurotrophin signalling is involved in the elevation of dendritic pS9-GSK3β levels. 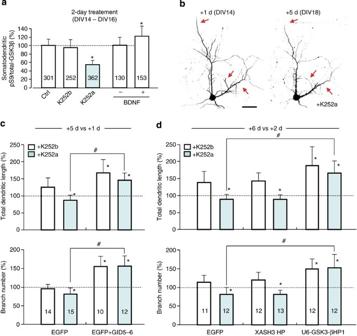Figure 2: Regulation of GSK3b activity and dendritic growth by neurotrophic factors. (a) Bar graph summarizes the effects of 2-day bath application of K252a (200 nM), K252b (200 nM) or BDNF (100 ng ml−1) on the pS9/Total-GSK3β ratio in the somatodendritic region. Numbers indicate the number of cells examined. (b) Representative confocal images of hippocampal neurons expressing EGFP treated with K252a, at 1 and 5 days post transfection. Arrows indicate shrinking dendritic branches. Scale bar, 50 μm. (c,d) Bar graphs show the normalized changes (+5 versus+1 d or +6 versus+2 d) in total dendritic length and branch number under different conditions. Numbers indicate the total number of cells examined (from at least three independent batches of culture). Error bars: s.d. *P<0.05 comparing with the EGFP K252b treated group,#P<0.05 comparing between the labelled groups (Student’st-test). Figure 2: Regulation of GSK3b activity and dendritic growth by neurotrophic factors. ( a ) Bar graph summarizes the effects of 2-day bath application of K252a (200 nM), K252b (200 nM) or BDNF (100 ng ml −1 ) on the pS9/Total-GSK3β ratio in the somatodendritic region. Numbers indicate the number of cells examined. ( b ) Representative confocal images of hippocampal neurons expressing EGFP treated with K252a, at 1 and 5 days post transfection. Arrows indicate shrinking dendritic branches. Scale bar, 50 μm. ( c , d ) Bar graphs show the normalized changes (+5 versus+1 d or +6 versus+2 d) in total dendritic length and branch number under different conditions. Numbers indicate the total number of cells examined (from at least three independent batches of culture). Error bars: s.d. * P <0.05 comparing with the EGFP K252b treated group, # P <0.05 comparing between the labelled groups (Student’s t -test). Full size image To examine the effects of neurotrophin signalling on dendrites, we transfected DIV13 hippocampal neurons with EGFP constructs and imaged the same EGFP-expressing neurons at 1 and 5 days post transfection (referred to as +1 d and +5 d). Cells were treated with K252a or K252b immediately after the initial imaging for the next 4 days, followed by imaging on +5 d. We found that neurons treated with K252a exhibited reduced dendritic growth and shrinkage of some dendritic branches (red arrows, Fig. 2b ). We quantified the total dendritic length and the number of dendritic braches on +1 d and +5 d and normalized these values (+5 d versus +1 d) to better illustrate the changes over the 4-day period. We found that neurons exposed to K252b, the ineffective compound, continued to extend their dendritic branches, resulting in an increase in the total dendritic length whereas the number of dendritic branches remained unchanged (mean±s.d. : 125.6±26.1% and 92.9±10.1% of the +1 d values, respectively, n =14) ( Fig. 2c ). However, inhibition of Trk receptors by K252a caused a marked reduction in total dendritic length and branch number (mean±s.d. : 86.8±13.9% and 80.9±16.0% of the +1 d values, respectively, n =15). Because K252a caused a substantial reduction in pS9-GSK3β levels, we suspected that K252a-induced dendritic reduction might be mediated by GSK3β activation. To test this possibility, we expressed GID5–6, an inhibitory peptide derived from the GSK3β binding domain of Axin [19] , [27] . We found that GID5-6 expression not only caused a marked increase in dendritic growth, but also abolished the dendritic reduction induced by K252a ( Fig. 2c ). To further confirm that GSK3β mediated K252a-induced reduction in dendritic growth, we used small hairpain RNA (shRNA) to specifically knock down GSK3β (U6-GSK-3βHP1) [28] . Immunostaining confirmed the effectiveness of GSK3β knockdown by this shRNA, but not the control shRNA (XASH3HP) ( Supplementary Fig. S3 ). To allow a sufficient time for shRNA-mediated knockdown of GSK3β, we examined the cells +2 d and +6 d after transfection. We found that GSK3β knockdown further enhanced the dendritic growth in this 4-day period in the presence of the ineffective K252b. Importantly, neurons expressing U6-GSK-3βHP1 showed substantial dendritic growth even after 4-day exposure to K252a, whereas cells expressing the control shRNA exhibited marked reduction in dendritic branches ( Fig. 2d ). These results suggest that neurotrophin-dependent dendritic growth and arborization are mediated by GSK3β inhibition in the somatodendritic region. To better understand how GSK3β activity regulates dendritic growth and arborization, we expressed a constitutively active GSK3β mutant, in which serine-9 was replaced with alanine (S9A). To minimize any potential effects on neuronal polarity and axonal development, hippocampal neurons were transfected at DIV13 with a plasmid encoding myc-tagged GSK3β-S9A, together with a plasmid encoding EGFP for visualization. Immunostaining showed that neurons expressing GSK3β-S9A exhibited a reduced level of pS9-GSK3β, indicating overall elevated GSK3β activity in these cells ( Supplementary Fig. S4 ). The dendrites of control EGFP-expressing neurons showed continuous, but small growth between DIV14 and DIV18 (green arrows, Fig. 3a ). However, hippocampal neurons expressing GSK3β-S9A underwent progressive shrinkage of their dendritic branches over the same time period (red arrows, Fig. 3a ). On the other hand, inhibition of GSK3β by GID5–6 promoted dendritic growth (green arrows, Fig. 3a ). Together, these results suggest that activation and inhibition of GSK3β cause dendritic shrinkage and growth, respectively. 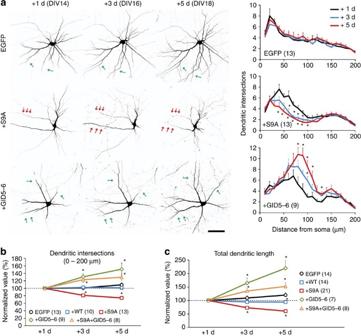Figure 3: Regulation of dendritic development by GSK3b. (a) Representative confocal images of hippocampal neurons expressing EGFP alone, GSK3β-S9A (+S9A) and GID5–6 (+GID5–6) at 1, 3 and 5 days after transfection. Images were inverted in grayscale for presentation. Red and green arrows indicate the shrinkage and growth of dendritic branches, respectively. Scale bar, 50 μm. The line graphs on the right depict the results of Sholl analysis. *P<0.05 (Student’st-test), comparing with +1 d. Numbers in brackets indicate the total number of cells examined (from at least three independent batches of culture). (b,c) Line graphs summarize the changes in dendritic intersections from the Sholl analysisband the total dendritic lengthcat different days after transfection. *P<0.05 (Student’st-test) comparing with the corresponding point of the EGFP group. For each condition, the data are normalized to the +1day. Each measure was from at least three independent cultures. Numbers in brackets indicate the total number of cells examined. Error bars represent the s.e.m. Figure 3: Regulation of dendritic development by GSK3b. ( a ) Representative confocal images of hippocampal neurons expressing EGFP alone, GSK3β-S9A (+S9A) and GID5–6 (+GID5–6) at 1, 3 and 5 days after transfection. Images were inverted in grayscale for presentation. Red and green arrows indicate the shrinkage and growth of dendritic branches, respectively. Scale bar, 50 μm. The line graphs on the right depict the results of Sholl analysis. * P <0.05 (Student’s t -test), comparing with +1 d. Numbers in brackets indicate the total number of cells examined (from at least three independent batches of culture). ( b , c ) Line graphs summarize the changes in dendritic intersections from the Sholl analysis b and the total dendritic length c at different days after transfection. * P <0.05 (Student’s t -test) comparing with the corresponding point of the EGFP group. For each condition, the data are normalized to the +1day. Each measure was from at least three independent cultures. Numbers in brackets indicate the total number of cells examined. Error bars represent the s.e.m. Full size image To quantify the effects of GSK3β on dendritic growth, we performed Sholl analysis [29] on neurons 1, 3 and 5 days after transfection. GSK3β-S9A expression significantly reduced the number of dendritic intersections between 20–100 μm radii, whereas EGFP alone had no effect (line plots in Fig. 3a ). Expression of the GSK3β inhibitor GID5–6 resulted in a marked increase in the number of dendritic intersections. To compare the changes in dendrites across different groups, we summed the dendritic intersections within a radius of 10–200 μm, as changes were mostly observed in this range. It is clear that 5 days after expression of GSK3β-S9A, the total number of dendritic intersections was reduced to 74.45±3.16% (mean±s.e.m., n =13) ( Fig. 3b ). Similarly, the total length of dendritic branches was reduced substantially by GSK3β-S9A expression, but not EGFP alone or wild-type GSK3β ( Fig. 3c ). Conversely, expression of GID5–6 promoted dendritic growth. Moreover, co-expression of GID5–6 with GSK3β-S9A effectively abolished S9A-induced dendritic reduction. Because over activation of GSK3β could induce neuronal apoptosis, we examined the viability of cells expressing GSK3β-S9A. We used Hoechst 33342 dye to identify apoptotic cells, and propidium iodide (PI) to stain dead cells. Neurons transfected with either EGFP alone or EGFP and GSK3β-S9A were live stained with Hoechst 33342 and PI 5 days post transfection. We found that GSK3β-S9A expression did not cause a significant increase in either cell apoptosis or cell death in our cultures ( Supplementary Fig. S5a,b ). To further exclude any non-specific effects from multi-day imaging, we also examined neurons after our five day imaging protocol, and found no effect on cell viability ( Supplementary Fig. S5c ). To confirm the role of GSK3β activity on dendrite growth and stability, we utilized organotypic hippocampal slice cultures. Biolistic gene gun transfection was used to deliver DNA constructs encoding EGFP, GSK3β-S9A and GID5–6 into cells in slices. For simplicity, we only analysed the apical dendrites of pyramidal neurons and summarized changes in the length of apical dendritic branches in composite drawings, with red segments indicating shrinkage and green segments representing growth ( Fig. 4a ). For neurons expressing EGFP alone, small changes in both directions (growth and shrinkage) in apical dendritic branches were observed. This is likely due to the fact that the hippocampal slices were derived from postnatal rats and the neurons are more mature and stable in comparison with the dissociated embryonic cultures. Consistent with our findings in the dissociated neurons, we found that over an 8-day period, GSK3β-S9A expression caused a substantial shrinkage of dendritic branches as highlighted by many red segments ( Fig. 4a ). Quantitative analysis confirmed that GSK3β-S9A caused a marked reduction in both the length and number of dendritic branches ( Fig. 4b ). Comparing +10 d to +2 d, the dendritic length and branch number were reduced to 75.6±17.1% and 82.7±15.2% (mean±s.d., n =5), respectively. However, expression of GID5-6 resulted in a small increase in both dendritic length and branch number (mean±s.d. : 108.4±8.6% and 109.1±2.9% of the +2 d values, respectively, n =3). These data thus indicate that dendritic effects of GSK3β are not an artifact of in vitro cell cultures. 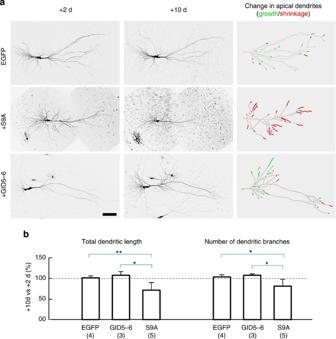Figure 4: Reduction in dendritic branches by GSK3b activation in organotypic hippocampal slices. (a) Representative two-photon confocal images of CA3 hippocampal neurons expressing EGFP alone, EGFP with GSK3β-S9A (S9A) and EGFP with GID5–6 (GID5–6) at 2 and 10 days after biolistic transfection. Images were inverted in grayscale for presentation. Composite tracings of the apical dendrites are shown on the right, with the red and green segments representing shrinkage and growth, respectively. Scale bar, 100 μm. (b) Bar graphs show changes in total dendritic length and branch number as labelled. For each condition, data are normalized to the 2 day after transfection values. Numbers in brackets indicate the number of cells examined (from at least three independent batches of culture). Error bars: s.d. *P<0.05 and **P<0.005 by Student’st-test. Figure 4: Reduction in dendritic branches by GSK3b activation in organotypic hippocampal slices. ( a ) Representative two-photon confocal images of CA3 hippocampal neurons expressing EGFP alone, EGFP with GSK3β-S9A (S9A) and EGFP with GID5–6 (GID5–6) at 2 and 10 days after biolistic transfection. Images were inverted in grayscale for presentation. Composite tracings of the apical dendrites are shown on the right, with the red and green segments representing shrinkage and growth, respectively. Scale bar, 100 μm. ( b ) Bar graphs show changes in total dendritic length and branch number as labelled. For each condition, data are normalized to the 2 day after transfection values. Numbers in brackets indicate the number of cells examined (from at least three independent batches of culture). Error bars: s.d. * P <0.05 and ** P <0.005 by Student’s t -test. Full size image We also confirmed the role of GSK3β in dendritic growth by using two pharmacological inhibitors of GSK3β. Bath application of either SB415286 (ref. 30 ) or CT99021 (ref. 31 ) promoted dendritic growth in EGFP-expressing cells, as well as alleviated GSK3β-S9A-induced dendritic shrinkage ( Supplementary Fig. S6a,b ). Furthermore, we found that knockdown of GSK3β by two different shRNAs (U6-GSK-3βHP1 and U6-GSK-3βHP2) largely enhanced dendrite extension, similar to the effect of GID5-6 expression ( Supplementary Fig. S6c ). Moreover, we observed that inhibition of PI-3 kinase by LY294002, which leads to GSK3β activation [19] , resulted in pronounced dendritic shrinkage, similar to the effect of GSK3β-S9A expression ( Supplementary Fig. S6d ). All together, these results suggest that the inhibition of GSK3β is required for normal dendritic growth and maintenance, whereas GSK3β activation leads to dendritic shrinkage. Neuronal activity mediates GSK3β-induced dendritic shrinkage We examined the role of neuronal activity in GSK3β-S9A-induced dendrite shrinkage. Inhibition of neuronal activity by tetrodotoxin (TTX) was found to enhance dendritic growth and, importantly, attenuate the dendritic shrinkage induced by GSK3β-S9A ( Fig. 5 ). Inhibition of NMDA receptors or AMPA receptors by APV or CNQX, respectively, was also effective in blocking the dendritic shrinkage in GSK3β-S9A-expressing neurons ( Fig. 5 ). These results suggest that the excitatory neuronal activity underlies the dendritic shrinkage induced by GSK3β activation. 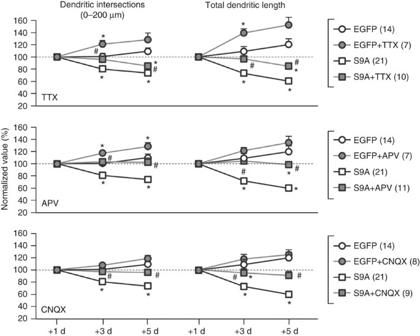Figure 5: Activity dependence of dendrite shrinkage induced by GSK3b-S9A expression. Number of dendritic intersections between 10–200 μm radii and total dendritic length are shown as normalized to the +1day values. Numbers in brackets indicate the total number of cells examined for each group (from at least three independent batches of culture). Error bars: s.e.m. *P<0.05 comparing with the corresponding point of the EGFP group (Student’st-test).#P<0.05 between GSK3β-S9A and GSK3β-S9A+inhibitors (TTX, APV or CNQX) groups (Student’st-test). Figure 5: Activity dependence of dendrite shrinkage induced by GSK3b-S9A expression. Number of dendritic intersections between 10–200 μm radii and total dendritic length are shown as normalized to the +1day values. Numbers in brackets indicate the total number of cells examined for each group (from at least three independent batches of culture). Error bars: s.e.m. * P <0.05 comparing with the corresponding point of the EGFP group (Student’s t -test). # P <0.05 between GSK3β-S9A and GSK3β-S9A+inhibitors (TTX, APV or CNQX) groups (Student’s t -test). Full size image To further test this hypothesis, we performed whole-cell voltage-clamp recording to examine how synaptic transmission is affected by GSK3β-S9A expression. We first recorded the miniature excitatory synaptic currents (mEPSCs) and found no significant difference in the frequency or amplitude of mEPSCs among the EGFP, WT-GSK3β, GSK3β-S9A and GID5–6-expressing neurons ( Fig. 6a ). Surprisingly, however, both the frequency and amplitude of miniature inhibitory synaptic currents (mIPSCs) were significantly reduced in the GSK3β-S9A-expressing neurons in comparison with EGFP-expressing neurons ( P <0.005, paired Student’s t -test, n =9). These results suggest that GSK3β-S9A expression in postsynaptic neurons did not affect the excitatory input, but instead reduced the strength of the inhibitory input these neurons received. As the overall activity of a neuron is controlled by a balance of excitatory and inhibitory inputs, a reduction in inhibitory strength should lead to an increase in overall neuronal excitability even in the absence of any changes in excitatory input. For simplicity, we tested this notion by measuring spontaneous postsynaptic currents (sPSCs) in the absence of TTX and other channel blockers to allow action potential-dependent neurotransmission. It should be noted that sPSCs represent integrated currents from both excitatory and inhibitory inputs. Moreover, it is well established that dendritic membrane expresses voltage-gated sodium and calcium channels and cannot be effectively voltage-clamped by the somatic clamping technique [32] , [33] . Therefore, sPSCs likely also contain contributions from voltage-gated channels on the dendritic surface. We found that GSK3β-S9A-expressing neurons displayed a higher frequency of sPSCs than neighbouring non-transfected neurons in the same network ( Fig. 6b ). These results support the notion that activated GSK3β reduces the inhibitory signalling to the neuron, leading to an increase in overall neuronal excitability and dendritic shrinkage. 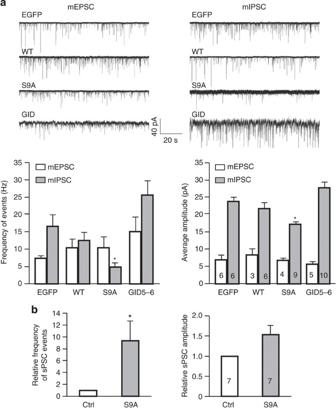Figure 6: Reduction of inhibitory synaptic strength by GSK3b activation. Whole-cell patch-clamp recordings showing the changes in postsynaptic currents in hippocampal neurons expressing EGFP, EGFP with wild-type GSK3β (WT), EGFP with GSK3β-S9A (S9A), and EGFP with GID5–6. Cells were transfected at DIV13 and recordings were performed between DIV17-19. (a) Measurements of the miniature excitatory and inhibitory postsynaptic currents. Sample traces of mEPSC and mIPSC are shown on the top and the quantified frequencies and amplitudes are shown in the bar graphs below. mIPSCs are inward at −80 mV becauseECl=0 mV. *P<0.05 comparing with the EGFP group (Student’st-test). (b) Bar graphs show the spontaneous postsynaptic currents (sPSCs) in neurons expressing GSK3β-S9A and normalized to neighbouring, non-transfected neurons (Ctrl). *P<0.05 comparing with the control group (Student’st-test). Numbers indicate the total number of cells examined for each group (from at least three independent batches of culture). Error bars: s.e.m. Figure 6: Reduction of inhibitory synaptic strength by GSK3b activation. Whole-cell patch-clamp recordings showing the changes in postsynaptic currents in hippocampal neurons expressing EGFP, EGFP with wild-type GSK3β (WT), EGFP with GSK3β-S9A (S9A), and EGFP with GID5–6. Cells were transfected at DIV13 and recordings were performed between DIV17-19. ( a ) Measurements of the miniature excitatory and inhibitory postsynaptic currents. Sample traces of mEPSC and mIPSC are shown on the top and the quantified frequencies and amplitudes are shown in the bar graphs below. mIPSCs are inward at −80 mV because E Cl =0 mV. * P <0.05 comparing with the EGFP group (Student’s t -test). ( b ) Bar graphs show the spontaneous postsynaptic currents (sPSCs) in neurons expressing GSK3β-S9A and normalized to neighbouring, non-transfected neurons (Ctrl). * P <0.05 comparing with the control group (Student’s t -test). Numbers indicate the total number of cells examined for each group (from at least three independent batches of culture). Error bars: s.e.m. Full size image Dendritic shrinkage arises from reduced GABA A R expression GABAergic synapses represent a major class of inhibitory synapses for hippocampal neurons [34] . We found that expression of GSK3β-S9A for 3–5 days led to a reduction in surface GABA A R levels compared with control neurons expressing EGFP ( Fig. 7a ). Conversely, expression of GID5–6 resulted in an increase in surface GABA A Rs. Quantification shows that expression of GSK3β-S9A and GID5–6 markedly reduced and increased the number and size of surface GABA A R puncta, respectively ( Fig. 7c,d ). In contrast, surface staining of the AMPA receptor subunit, GluA1, was unchanged under identical conditions ( Fig. 7b,e,f ). These findings support our electrophysiology data, and suggest that GABA receptors of inhibitory synapses, but not glutamate receptors of excitatory synapses, are the target of dendritic GSK3β activity. 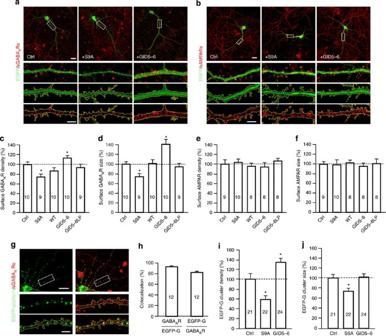Figure 7: Regulation of surface GABAAreceptors by GSK3b activation. (a,b) Representative images show surface GABAARs by γ2 staining (a) and AMPARs by GluA1 labelling (b) on dendrites of neurons expressing EGFP (Ctrl), GSK3β-S9A (+S9A) and GID5-6 (+GID5-6) at DIV16 (+3 d after transfection). Dendritic regions enclosed by the white rectangles in the top panels are shown in magnified views below. For each cell, three high magnification panels are shown: colour merged (green: EGFP, red: surface receptors), EGFP with yellow outline of the dendritic segment, and surface GABAAreceptors with regions outside of dendritic segment masked using EGFP fluorescence. Scale bar in top panels, 20 μm, lower panels, 5 μm. (c,d) Bar graphs show changes in density and size of surface GABAAR puncta normalized to the EGFP group (Ctrl). (e,f) Bar graphs show the normalized changes in density and size of AMPAR puncta. (g) Representative images show the co-localization of EGFP-gephyrin clusters with surface GABAARs. Magnified panels are shown below. Scale bars are 20 μm and 5 μm for the top and bottom panels, respectively. (h) Bar graph depicts incidents of co-localization between EGFP-gephyrin (EGFP-G) and surface GABAARs. The first bar indicates the percentage of EGFP-G puncta colocalized with GABAAR clusters, and the second represents the percentage of GABAAR clusters localized with EGFP-G puncta on the same branch. (i,j) Bar graphs depict the changes in density and size of EGFP-gephyrin puncta in dendrites at DIV16 (+3 after transfection). Numbers indicate the total number of cells examined for each group (from at least three independent batches of culture). Error bars: s.e.m. *P<0.05 compared with EGFP-G (Ctrl) by Student’st-test. Figure 7: Regulation of surface GABA A receptors by GSK3b activation. ( a , b ) Representative images show surface GABA A Rs by γ2 staining ( a ) and AMPARs by GluA1 labelling ( b ) on dendrites of neurons expressing EGFP (Ctrl), GSK3β-S9A (+S9A) and GID5-6 (+GID5-6) at DIV16 (+3 d after transfection). Dendritic regions enclosed by the white rectangles in the top panels are shown in magnified views below. For each cell, three high magnification panels are shown: colour merged (green: EGFP, red: surface receptors), EGFP with yellow outline of the dendritic segment, and surface GABA A receptors with regions outside of dendritic segment masked using EGFP fluorescence. Scale bar in top panels, 20 μm, lower panels, 5 μm. ( c , d ) Bar graphs show changes in density and size of surface GABA A R puncta normalized to the EGFP group (Ctrl). ( e , f ) Bar graphs show the normalized changes in density and size of AMPAR puncta. ( g ) Representative images show the co-localization of EGFP-gephyrin clusters with surface GABA A Rs. Magnified panels are shown below. Scale bars are 20 μm and 5 μm for the top and bottom panels, respectively. ( h ) Bar graph depicts incidents of co-localization between EGFP-gephyrin (EGFP-G) and surface GABA A Rs. The first bar indicates the percentage of EGFP-G puncta colocalized with GABA A R clusters, and the second represents the percentage of GABA A R clusters localized with EGFP-G puncta on the same branch. ( i , j ) Bar graphs depict the changes in density and size of EGFP-gephyrin puncta in dendrites at DIV16 (+3 after transfection). Numbers indicate the total number of cells examined for each group (from at least three independent batches of culture). Error bars: s.e.m. * P <0.05 compared with EGFP-G (Ctrl) by Student’s t -test. Full size image To verify that our GABA A R staining faithfully reported surface GABA A R clusters, we stained surface GABA A R clusters in neurons expressing EGFP-gephyrin, a scaffold protein that mediates GABA A R surface clustering. Our data show that 93.3±4.6% (mean±s.e.m., n =12) of EGFP-gephyrin puncta colocalized with surface GABA A R puncta, indicating that the staining reliably detects surface GABA A R clusters ( Fig. 7g,h ). Consistent with our GABA A R staining, we found that neurons expressing GSK3β-S9A caused a reduction in the density and size of EGFP-gephyrin puncta in dendrites, whereas GID5–6 increased the density of EGFP-gephyrin puncta, but not their size ( Fig. 7i,j ). We also stained surface GluA1 receptors in neurons expressing EGFP-gephyrin to further confirm that GSK3β-S9A does not affect surface GluA1 in the same dendritic branches ( Supplementary Fig. S7 ). These data are consistent with the electrophysiological recordings, and suggest that GSK3β activation selectively targets inhibitory synapses by reducing surface GABA A Rs. To determine if reduced GABAergic activity is the cause of GSK3β activation-induced dendritic shrinkage, we examined dendritic growth in the presence of GABA A R agonists or antagonists. We found that the GABA A R agonist muscimol significantly increased dendritic growth ( Fig. 8a ), whereas the antagonist picrotoxin caused dendritic shrinkage ( Fig. 8b ). Interestingly, muscimol was unable to attenuate the dendritic shrinkage induced by GSK3β-S9A expression, suggesting that the number of surface GABA A Rs is the determinant factor. We next performed knockdown experiments using shRNAs against the 3′-untranslated region (UTR) of the GABA A R γ2 subunit (γ2 UTR), or a scrambled control shRNA (γ2 UTR3m) [35] . Hippocampal neurons were cotransfected with the shRNA and EGFP constructs on DIV13, and fixed 5 days later. We found that γ2 UTR resulted in a marked reduction of surface GABA A R puncta and gephyrin clusters [35] , whereas γ2 UTR3m had no effect ( Fig. 8c ). Importantly, γ2 knockdown resulted in marked dendritic shrinkage, similar to that of GSK3β-S9A expression, whereas the control shRNA had no effect ( Fig. 8d ). Quantitative analysis showed that GABA A R knockdown resulted in a decline in dendritic complexity, similar to that of GSK3β-S9A expression. Expression of the GSK3β inhibitor peptide GID5–6, however, was unable to rescue the dendritic shrinkage induced by GABA A R knockdown, suggesting that GSK3β acts upstream of GABA A Rs. Together, these findings suggest that GSK3β inhibition is required for the presence of GABA A Rs on the neuronal cell surface. 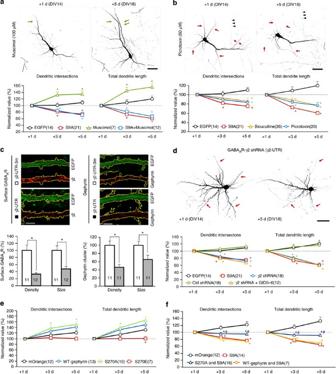Figure 8: Effects of GABAAR manipulations on dendritic development. (a,b) Effects of GABAAR agonist and antagonist on dendrites. Hippocampal neurons were transfected on DIV 13, and treated with either Muscimol (GABAAR agonist) (a) or Picrotoxin and bicuculline (GABAAR antagonists) (b) after initial imaging on DIV 14 (+1 d). Representative images of EGFP-expressing neurons are shown on the top. Green and red arrows indicate the growth and shrinkage of dendritic branches, respectively. Normalized number of dendritic intersections and total length are shown at the bottom. Scale bars, 50 μm. *P<0.05 comparing with the corresponding point of EGFP-expressing cells (Student’st-test). (c,d) Effects of GABAAR knockdown on dendrite development. (c) Neurons transfected with shRNAs were identified by EGFP fluorescence. Representative confocal images of EGFP fluorescence and immunofluorescence (of GABAAR or gephyrin) are shown on top. Scale bars=5 μm. The bar graphs show the cluster size and density of surface GABAAR (left) and cytoplasmic gephyrin (right) in cells expressing the shRNA (r2-UTR) or the control shRNA (r2-UTR-3m). *P<0.01, Student’st-test. (d) GABAAR knockdown results in dendritic shrinkage. Representative images of EGFP-expressing neurons are shown at the top. Scale bar, 50 μm. Normalized number of dendritic intersections and total length are shown at the bottom. For each group, all data are normalized to the +1 day. *P<0.05 comparing with the corresponding point of the control (EGFP, Student’st-test). (e,f) Effects of co-expression of wild–type gephyrin, S270A-gephyrin and S270E-gephyrin, without (e) or with (f) GSK3β-S9A on dendrites. The line graphs show the number of dendritic intersections and total dendritic length. *P<0.05 comparing to the corresponding point of the mOrange group (Student’st-test).#P<0.05 comparing with the corresponding point of GSK3β-S9A group (Student’st-test). The data are normalized to +1 d. Numbers in brackets indicate the number of cells examined for each group (from at least three independent batches of culture). Error bars: s.e.m. Figure 8: Effects of GABA A R manipulations on dendritic development. ( a , b ) Effects of GABA A R agonist and antagonist on dendrites. Hippocampal neurons were transfected on DIV 13, and treated with either Muscimol (GABA A R agonist) ( a ) or Picrotoxin and bicuculline (GABA A R antagonists) ( b ) after initial imaging on DIV 14 (+1 d). Representative images of EGFP-expressing neurons are shown on the top. Green and red arrows indicate the growth and shrinkage of dendritic branches, respectively. Normalized number of dendritic intersections and total length are shown at the bottom. Scale bars, 50 μm. * P <0.05 comparing with the corresponding point of EGFP-expressing cells (Student’s t -test). ( c , d ) Effects of GABA A R knockdown on dendrite development. ( c ) Neurons transfected with shRNAs were identified by EGFP fluorescence. Representative confocal images of EGFP fluorescence and immunofluorescence (of GABA A R or gephyrin) are shown on top. Scale bars=5 μm. The bar graphs show the cluster size and density of surface GABA A R (left) and cytoplasmic gephyrin (right) in cells expressing the shRNA (r2-UTR) or the control shRNA (r2-UTR-3m). * P <0.01, Student’s t -test. ( d ) GABA A R knockdown results in dendritic shrinkage. Representative images of EGFP-expressing neurons are shown at the top. Scale bar, 50 μm. Normalized number of dendritic intersections and total length are shown at the bottom. For each group, all data are normalized to the +1 day. * P <0.05 comparing with the corresponding point of the control (EGFP, Student’s t -test). ( e , f ) Effects of co-expression of wild–type gephyrin, S270A-gephyrin and S270E-gephyrin, without ( e ) or with ( f ) GSK3β-S9A on dendrites. The line graphs show the number of dendritic intersections and total dendritic length. * P <0.05 comparing to the corresponding point of the mOrange group (Student’s t -test). # P <0.05 comparing with the corresponding point of GSK3β-S9A group (Student’s t -test). The data are normalized to +1 d. Numbers in brackets indicate the number of cells examined for each group (from at least three independent batches of culture). Error bars: s.e.m. Full size image Serine-270 of gephyrin was identified as a target of GSK3β, and shown to modulate gephyrin clustering and GABAergic synaptic transmission [36] . We thus expressed a phosphorylation defective S270A-gephyrin mutant and a phospho-mimetic S270E-gephyrin mutant. We found that expression of the S270A mutant slightly increased dendrite growth, whereas expression of the S270E mutant slightly decreased dendrite growth ( Fig. 8e ). Importantly, however, co-expression of the S270A-gephyrin mutant with GSK3β-S9A, but not wild-type gephyrin, was able to attenuate GSK3β-S9A-induced dendrite shrinkage ( Fig. 8f ). These findings suggest that GSK3β controls dendritic growth by regulating surface GABAR clustering through phosphorylation of gephyrin at serine-270. The highly elaborate dendritic arbours of a neuron host a large number of synapses that are organized in spatial domains for distinct synaptic inputs [37] . Their proper development and maintenance are crucial for the reception, integration and computation of synaptic signals that encode spatial and temporal information. It is well established that genetic programming, neuronal activity and extracellular factors work in concert to shape dendritic arbourization patterns [3] , [4] . Synaptic activity is also believed to have an important role in the stabilization of dendritic arbours. Individual dendritic arbours are often maintained for up to decades, and their disruption has been observed in many neurological diseases [8] , [9] . Although activity-dependent dendritic growth and stabilization represent a key step of dendrite development, the molecular and cellular mechanisms that translate neuronal activities into distinct dendritic outputs currently remain unknown. In this study, we have identified an important role for GSK3β in activity-dependent dendrite growth and stabilization. Our findings reveal an intriguing mechanism in which GSK3β targets the surface levels of GABA A Rs to regulate the balance of neuronal excitation and inhibition to control dendritic growth. Importantly, we show that activation of GSK3β results in a reduction of GABAergic signalling via phosphorylation of the scaffold protein gephyrin, leading to dendrite atrophy. Our results thus provide important insights into the mechanisms of activity-dependent dendrite development and maintenance. GSK3β is known for its role in axonal specification during development [19] . It remains unclear, however, how spatially restricted GSK3β phosphorylation is achieved for polarity formation. Growth factors have been suggested to locally activate PI-3 kinase and Akt/PKB to inhibit GSK3β by phosphorylation [10] . Previous studies have shown that expression of two neurotrophins, BDNF and NT-3, are elevated upon synaptogenesis, and that both neurotrophins have a role in dendrite development [25] . Furthermore, a BDNF knockout mouse displayed reduced dendritic arborization, supporting a role for neurotrophins in dendrite development [38] . In this study, we show that GSK3β serine-9 phosphorylation in somatodendric regions was substantially elevated at DIV9 and later stages, likely in correspondence with synapse formation and maturation. This increase in serine-9 phosphorylation is at least partly a result of neurotrophin signalling, as inhibition of Trk receptors by K252a substantially reduced the pS9-GSK3β level in dendrites, whereas exogenous BDNF treatment increased pS9-GSK3β levels. Whether other members of the neurotrophin family are involved in GSK3β serine-9 phosphorylation remains to be determined. Nonetheless, inhibition of Trk receptors resulted in a reduction in dendritic arborization, which was blocked by inhibition or knockdown of GSK3β. These results connect neurotrophin signalling to GSK3β in regulating dendritic growth. It is conceivable that elevated expression and secretion of neurotrophic factors upon synaptogenesis elicit S9 phosphorylation of GSK3β in dendrites, which in turn enhances dendrite development. The functional consequence of increased GSK3β inhibition via serine-9 phosphorylation in the somatodendritic region appears to enable dendritic growth and stabilization. We found that activation of GSK3β causes dendrite atrophy, whereas inhibition results in enhanced extension of dendritic branches. It should be noted that these studies do not preclude a similar role for the GSK3β homologue, GSK3α, in dendritic development and maintenance. The kinase domains of both GSK3α and GSK3β are highly similar, and there are numerous contexts where both have been demonstrated to be at least partially functionally redundant [39] , [40] . Our data show that GSK3β targets the surface levels of GABA A receptors to selectively modulate the balance between excitatory and inhibitory inputs on the dendrites. By tilting the balance to increased neuronal excitation, dendrite shrinkage was favored. Consistent with this result, hyperexcitability from chronic inhibition of GABAergic transmission was found to reduce dendritic length of CA1 hippocampal pyramidal neurons in slice culture [41] . Therefore, a balancing act of excitatory and inhibitory activities appears to be a key component of activity-dependent regulation of dendritic development and maintenance. Our conclusion that GSK3β mainly targets the surface expression of GABA A receptors to affect dendritic branches is based on several lines of experiments: (1) electrophysiology data showed a substantial reduction of mIPSCs by GSK3β-S9A expression, without effects on mEPSCs; (2) quantitative immunofluorescence showed the reduction of surface GABA A Rs without changes in AMAPRs; (3) GABA A R antagonists mimicked the dendritic shrinkage induced by GSK3β-S9A; (4) knockdown of GABA A Rs reproduced the dendritic shrinkage phenotype; (5) gephyrin S270A mutant could attenuate GSK3β-S9A-induced dendritic shrinkage. It should be noted that inhibition of GSK3β by GID5–6 was unable to attenuate the dendrite shrinkage induced by GABA A R knockdown, supporting the notion that GSK3β acts upstream of GABA A Rs. The finding that GABA A R agonist muscimol was unable to rescue the effects induced by GSK3β-S9A expression suggests that further activation of the reduced number of GABA A Rs may not be sufficient to restore the strength of inhibitory inputs. Previous studies have shown that GSK3β phosphorylates gephyrin, a key scaffolding protein for the localization and accumulation of GABA A Rs at the postsynaptic surface of inhibitory synapses [36] , [42] . It is plausible that gephyrin is involved in the GSK3β regulation of dendritic development through GABA A Rs. Indeed, we found that gephyrin puncta in dendrites were substantially reduced and increased by GSK3β-S9A and GID5–6 expression, respectively ( Fig. 7i,j ). We further confirmed that gephrin is involved in GSK3β-S9A-induced dendritic shrinkage as S270A-gephyrin mutant, which cannot be phosphorylated by GSK3β, blocked the dendritic reduction by GSK3β-S9A. Dendrite atrophies have been observed in a wide range of neurological disorders ranging from Alzheimer’s disease to Schizophrenia [8] . Dendrite abnormality is the strongest correlate with mental retardation [3] . However, the mechanisms leading to the alteration of dendritic arbours in specific diseases remain to be elucidated. Interestingly, both aberrantly elevated GSK3β activity and reduced GABAergic synaptic signalling have been associated with many, if not all of the neurological disorders, in which dendrite atrophy was observed, including Fragile X syndrome and FMR1 (refs 43 , 44 , 45 , 46 , 47 , 48 , 49 , 50 ). In addition, several signalling pathways upstream of GSK3β, including Akt and DISC1, have also been implicated in a large number of neurological disorders [10] , [15] , [16] , [18] , [51] . The findings in this study provide evidence that GSK3β activity, GABAergic signalling, and dendritic development and maintenance are ultimately connected. Alterations in this intricately connected pathway may lead to dendritic defects. Aberrantly elevated GSK3β activity could disrupt GABAergic signalling and alter the excitatory–inhibitory balance, resulting in dendritic atrophy and synapse loss. Therefore, the GSK3β–GABA A R–dendrite pathway may represent an important link that contributes to the structural and functional abnormality in brain disorders. DNA constructs and chemical reagents DNA constructs encoding wild-type GSK3β, GSK3β-S9A, Axin GID5–6, Axin GID5–6LP, XASH3HP, U6-GSK-3βHP1 and U6-GSK-3βHP2 were generously provided by Dr Yi Rao at Peking University, China [19] . pEGFP-C1 was purchased from Clontech. The small shRNA (γ2 UTR): 5′- GGUGAGAUUCAGCGAAUAAGACCCCUA-3′ targeted a sequence of the 3′UTR of the rat γ2 subunit (nucleotides 1,467–1,491); the control small shRNA (γ2 UTR3m): 5′-GGUGACAUACACCGAAUAAGACCCCUA-3′ was generated by introducing three point mutations in the sense and antisense arms of the corresponding shRNA [35] . EGFP-gephyrin was from rat gephyrin P1 variant cloned using EcoRI–KpnI sites and inserted to the carboxy-terminal of pEGFP-C2 construct. S270A-gephyrin and S270E-gephyrin mutants were made by mutating serine-270 to alanine or glutamate by a site-directed mutagenesis. We used the following antibodies and chemicals for our study: mouse anti-MAP2 (Sigma; 1:250), rabbit anti-MAP2 (EMD Millipore; 1:2,000), mouse anti-total-GSK3β (Abcam; 1:500), rabbit anti-pS9-GSK3β (Cell Signaling; 1:50), mouse anti-pY216-GSK3β (BD Biosciences; 1;200), rabbit anti-pY216-GSK3β (Abcam; 1:200), rabbit anti-GABA A R-γ2 (EMD Millipore; 1:300), rabbit anti-GluR1(EMD Millipore; 1:50), mouse anti-gephyrin (Synaptic system; 1:300), mouse anti-c-myc (Santa Cruz; 1:1,000) and mouse anti-HA (Santa Cruz; 1:200). SB415286, Muscimol was from Tocris; Ly294002 was from EMD Millipore; CT99021 was from Selleckchem; K252a, K252b, TTX, APV, CNQX, Bicucullin and picrotoxin were from Sigma; Hoechst 33342 was from Invitrogen and propidium iodide was from Abcam. Neuronal culture and transfection Sprague–Dawley timed-pregnant adult rats (8–10 weeks) were purchased from Charles River Laboratories. Primary hippocampal neurons were prepared from embryonic day 18 rat embryos and plated on 25-mm coverslips or 35-mm glass bottom dishes pretreated with 0.1 mg ml −1 poly- D -lysine (EMD Millipore) at a density of approximately 350,000 cells per dish [52] . Neurons were plated and maintained in Neurobasal medium supplemented with B-27 and GlutaMax (Invitrogen). Cells were transfected with a Calphos calcium phosphate transfection kit (Clontech) on DIV13 and imaged at different days after transfection. Each experiment was repeated at least three times from independent batches of cultures. All the experiments were carried out in accordance to the guidelines of US National Institutes of Health for animal use and were approved by the Institutional Animal Care and Use Committee of Emory University. Live-cell imaging For multi-day live-cell imaging of dendrite development, neurons cultured on glass-bottomed dishes were changed from normal culture medium to phenol-red free neurobasal medium and sealed with Parafilm. The sealed dish was placed on the microscope stage and housed in a temperature controlled chamber (Warner Instruments, New Haven, CT) at ~35 °C. Cells were imaged using a Nikon C1 laser-scanning confocal system based on a Nikon inverted microscope (TE300), with a 40 × N.A.1.3 Plan Fluor oil immersion objective. To image all of the dendritic branches at different focusing planes of a dendritic segment, z-stacks of images of EGFP-expressing neurons were acquired and converted to 2-dimensional images by maximal intensity projection. After imaging, the dish was unsealed, changed back to the original neurobasal medium, and returned to the CO 2 incubator for further culture and imaging at later time points. Organotypic hippocampal slice culture and imaging Hippocampal slice cultures were prepared from postnatal day 6 (P6) Sprague–Dawley rat pups (mixed sex) as previously described [53] . Briefly, rat pups were anesthetized and decapitated according to institutional guidelines, and then hippocampi were removed and transversely sliced (400-μm thick) using a McIlwain Tissue Chopper (Ted Pella, Inc). Slices were transferred onto 0.4 μm Millicell cell culture membrane inserts (Millipore) and cultured for 2 weeks. Biolistic transfection of neurons in hippocampal slices was then performed using a Helios gene gun (Bio-Rad) [54] . Cell imaging was performed using a two-photon FV1000 laser-scanning confocal (Olympus) 48 h after transfection, and again 10 days after transfection. CA3 pyramidal neurons expressing EGFP were randomly chosen by location and morphology. Maximal intensity projections of z-stacks were used to generate two-dimensional images for analysis. Tracing and quantification of dendrites were done using the Simple Neurite Tracer ImageJ plugin [55] . Electrophysiology Whole-cell patch-clamp recordings were performed using EPC7 amplifier (HEKA) as described previously [52] . Patch pipettes were pulled from borosilicate glass and fire polished (4–6 MΩ). The recording chamber was continuously perfused with HEPES buffered recording solution (128 mM NaCl, 5 mM KCl, 2 mM CaCl 2 , 1 mM MgCl 2 , 25 mM HEPES, 30 mM glucose, pH 7.3 adjusted with NaOH and osmolarity at 310–320 mOsmol −1 ). The pipette solution contained 147 mM KCl, 2 mM KH 2 PO 4 , 5 mM Tris-HCl, 2 mM EGTA, 10 mM HEPES, 4 mM Mg-ATP, 0.5 mM Na 2 GTP, pH 7.3 adjusted with KOH, and osmolarity at 310–320 mOsm (ref. 1 ). The membrane potential was clamped at −80 mV. Data were acquired using pClamp 9 software, sampled at 5 kHz and filtered at 1 kHz. For mEPSC recordings, 0.5 μM TTX and 20 μM bicuculline (or 100 μM picrotoxin) were added to block action potentials and GABA A receptors. For mIPSC recording, 0.5 μM TTX, 50 μM APV and 20 μM CNQX were added to block action potentials and NMDA and AMPA receptors. Here mIPSCs were inward at −80 mV as the reversal potential for Cl − was 0 mV. For recording of spontaneous PSCs (sPSCs), the pipette solution contained 140 mM K-gluconate, 2 mM MgCl 2 , 1 mM CaCl 2 , 11 mM EGTA, 10 mM HEPES, 2 mM Mg-ATP, 0.5 mM Na 2 GTP, pH 7.3 adjusted with N -methyl- D -glucamine, and osmolarity at 308 mOsm −1 . The cells were in normal recording buffer without channel blockers added. As a result, the reversal potential for Cl − was −79 mV. The cell was voltage clamped at −70 mV for recording sPSCs. Off-line data analysis of sPSC was performed using Clampfit 9.0 software (Molecular Devices). Data were expressed as mean±standard error of the mean. Paired Student’s t- test was used for testing statistical significance, unless otherwise stated. Analysis of dendrites We used the maximal intensity projection of z-stacks of images to generate the two-dimensional images for analysis. Tracing and quantification of dendrites were done using ImageJ with the NeuronJ plugin [56] . Only neurons showing intact dendritic arbourization were analysed and only branches over 10 μm in length were quantified. Sholl analysis was performed using ImageJ with the Sholl analysis plugin developed by the Ghosh Lab ( http://biology.ucsd.edu/labs/ghosh/software ) with a 10-μm interval in radius between concentric circles. Immunostaining For immunostaining of the total GSK3β and phospho-GSK3β (pS9 and pY216), neurons were fixed with 4% (w/v) paraformaldehyde containing 4% (w/v) sucrose in phosphate-buffered saline (PBS) for 20 min at room temperature. Fixed neurons were washed with PBS and blocked with 2% BSA (w/v) in cytoskeleton buffer (10 mM MES (pH 6.1), 138 M KCl, 3 m MgCl2, 2 m EGTA) [57] containing 0.1% (v/v) Triton X-100 at room temperature for 1 h. Then cells were incubated with primary antibodies overnight at 4 °C, followed by 1-h labelling with fluorescent secondary antibodies at room temperature. Both primary antibodies and secondary antibodies were diluted with the blocking buffer. For fluorescent staining of surface GABA A receptors and AMAP receptors, anti-γ2 subunit of GABA A Rs and anti-GluA1 subunit of AMPARs were incubated with live cells in Krebs-Ringer’s saline (KRB: 150 mM NaCl, 5 mM KCl, 2 mM CaCl 2 , 1 mM MgCl 2 , 10 mM glucose, and 10 mM HEPES, pH 7.4) for 20 min at 37 °C. The cells were then washed with PBS and fixed with 4% paraformaldehyde PBS for 20 min, followed by labelling with appropriate secondary antibodies in 1% BSA (w/v) for 45 min. For all other staining, neurons were fixed for 20 min with 4% (w/v) paraformaldehyde and permeabilized with 0.1% (w/v) Triton X-100 in PBS. After blocking with 3% (w/v) BSA in PBS for 1 h, cells were incubated with primary antibodies in blocking buffer overnight at 4 °C, followed by 1-h labelling with fluorescent secondary antibodies in 1% BSA (w/v) in PBS at room temperature. Cell death and viability assays Hippocampal neurons transfected with EGFP or GSK3β-S9A were incubated with 10 μM Hoechst 33342 dye and 5 μM PI in Kreb-Ringer’s buffer (KRB) at 37 °C for 15 min. Afterwards, the cells were washed three times with KRB buffer and imaged immediately. Western blotting Hippocampal neurons at DIV3, DIV9 and DIV16 under the same culture condition were collected, respectively. Cells were lysed using a lysis buffer containing 50 mM Tris-HCl (Ph 7.4), 150 mM NaCl, 1 mM ethylene diamine tetra-acetic acid (EDTA), 0.5% NP-40, 0.25% Na deoxycholate and 1 mM dithiothreitol (DTT), supplemented with 1 mM phenylmethylsulfonyl fluoride, protein inhibitor cocktail (Sigma, 1:100), 5 mM NaF and 2 mM Na 3 VO 4 . Bradford assay was used to quantify the total protein volume in each sample and 10 μg samples were added to NuPage sample buffer (Invitrogen) with 50 mM DTT and heated at 85 °C for 5 min. Samples were loaded and fractioned by SDS-PAGE on 10% Tris-glycine gel (Invitrogen) and subsequently transferred to nitrocellulose membranes for blotting. Antibodies used: mouse anti-GSK3β (Abcam, 1:2,000) and rabbit anti-pS9-GSK3β (Cell Signalling, 1:1,000). How to cite this article: Rui, Y. et al . Activity-dependent regulation of dendritic growth and maintenance by glycogen synthase kinase 3β. Nat. Commun. 4:2628 doi: 10.1038/ncomms3628 (2013).